A critical transition in leaf evolution facilitated the Cretaceous angiosperm revolution The revolutionary rise of broad-leaved (flowering) angiosperm plant species during the Cretaceous initiated a global ecological transformation towards modern biodiversity. Still, the mechanisms involved in this angiosperm radiation remain enigmatic. Here we show that the period of rapid angiosperm evolution initiated after the leaf interior (post venous) transport path length for water was reduced beyond the leaf interior transport path length for CO 2 at a critical leaf vein density of 2.5–5 mm mm −2 . Data and our modelling approaches indicate that surpassing this critical vein density was a pivotal moment in leaf evolution that enabled evolving angiosperms to profit from developing leaves with more and smaller stomata in terms of higher carbon returns from equal water loss. Surpassing the critical vein density may therefore have facilitated evolving angiosperms to develop leaves with higher gas exchange capacities required to adapt to the Cretaceous CO 2 decline and outcompete previously dominant coniferous species in the upper canopy. Almost 90% of present-day terrestrial plant biodiversity consists of flowering (angiosperm) species [1] . This ecological success of angiosperms did not grow gradually, rather, angiosperms so suddenly dominated the fossil record of the Cretaceous period between 145 and 66 million years (Ma) ago that even Charles Darwin found it challenging to his ideas on gradual evolution [2] , [3] . Evidence is now emerging that ancestral angiosperms existed in low evaporative niches during the Early Cretaceous [4] , [5] before the period of their rapid diversification in the Mid Cretaceous [6] . During the Late Cretaceous, evolving angiosperms spread poleward [7] and gained ecological dominance in most of the world’s ecosystems by replacing needle-leaved (gymnosperm) conifer tree species in the evaporatively more demanding upper canopy [8] ( Fig. 1a ). Previous explanations for this angiosperm radiation [1] include coevolution with insects [9] and positive environmental feedbacks [10] . Recent insights [11] suggest that the evolution towards more reticulated leaf venation [12] , [13] was linked to the escalation of angiosperm leaf gas exchange capacity [14] , [15] in relation to falling atmospheric CO 2 concentrations ( C a ) [16] , [17] during this floral regime shift. The resulting rise in productivity likely enabled evolving angiosperms to outcompete conifers in the upper canopy [18] . However, the underlying mechanisms involved in this angiosperm revolution remain unrevealed. 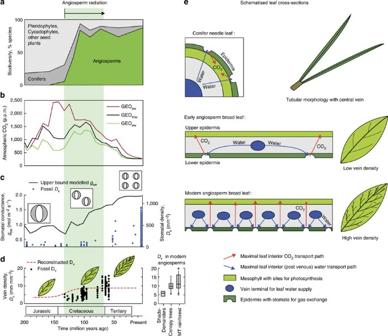Figure 1: Radiation of angiosperm plant species during the Cretaceous. (a) The angiosperm radiation occurred at the expense of pteridophytes (horsetails, ferns) and cycadophytes (cycades) living near the forest floor and conifers dominating the upper canopy1,6,7,8. (b) ModelledCafrom the GEOCARBSULF model51with parameterisations for standard (GEOsw), moderate (GEOmw) and enhanced (GEOew) volcanic weathering rates, following Fletcheret al.17(c) FallingCalikely drove leaf evolution towards higher stomatal gas exchange capacity via decreasing pore size and rising stomatal density (Ds)19,24. Data points indicate observations of fossilDs24, the black line indicates the upper bound on modelled stomatal conductance to water vapour (gsw)19. (d) Rising angiosperm leaf vein density (Dv) obtained from fossil leaves15and age-calibrated ancestral-state analyses14. The dashed sigmoid curve is based on the equation:Dv=3.3+5.3/(1+e−(time −130)/−8.7) following Brodribbet al.14In this equation the parameter ‘time’ is time in million years BP. Also indicated are ranges of modern angiospermDvfor woody shade demanders, canopy trees and for trees in megathermal rain forests, following Feildet al.15(e) Schematised cross-sections of a conifer needle leaf (top), an early hypostomatous angiosperm broad leaf (middle) with lowDvand lowDs, and a modern hypostomatous angiosperm broad leaf (bottom) with highDvand highDs. Figure 1: Radiation of angiosperm plant species during the Cretaceous. ( a ) The angiosperm radiation occurred at the expense of pteridophytes (horsetails, ferns) and cycadophytes (cycades) living near the forest floor and conifers dominating the upper canopy [1] , [6] , [7] , [8] . ( b ) Modelled C a from the GEOCARBSULF model [51] with parameterisations for standard (GEO sw ), moderate (GEO mw ) and enhanced (GEO ew ) volcanic weathering rates, following Fletcher et al . [17] ( c ) Falling C a likely drove leaf evolution towards higher stomatal gas exchange capacity via decreasing pore size and rising stomatal density ( D s ) [19] , [24] . Data points indicate observations of fossil D s [24] , the black line indicates the upper bound on modelled stomatal conductance to water vapour ( g sw ) [19] . ( d ) Rising angiosperm leaf vein density ( D v ) obtained from fossil leaves [15] and age-calibrated ancestral-state analyses [14] . The dashed sigmoid curve is based on the equation: D v =3.3+5.3/(1+e −(time −130)/−8.7 ) following Brodribb et al . [14] In this equation the parameter ‘time’ is time in million years BP. Also indicated are ranges of modern angiosperm D v for woody shade demanders, canopy trees and for trees in megathermal rain forests, following Feild et al . [15] ( e ) Schematised cross-sections of a conifer needle leaf (top), an early hypostomatous angiosperm broad leaf (middle) with low D v and low D s , and a modern hypostomatous angiosperm broad leaf (bottom) with high D v and high D s . Full size image Falling atmospheric CO 2 concentrations ( C a ) before and during the angiosperm radiation [16] , [17] ( Fig. 1b ) likely put evolutionary pressure on terrestrial C3 plants [19] because carbon uptake for photosynthesis is intrinsically linked to transpirative water loss through the stomatal pores on their leaf surfaces [20] . Natural selection may therefore have favoured those species with most plastic stomatal traits [21] , [22] capable of optimizing photosynthesis with minimal transpiration [19] , [23] . Consequentially, falling C a drove leaf evolution towards higher maximal stomatal conductance ( g smax ) [24] ( Fig. 1c ). The exchange of water vapour for CO 2 through stomata is principally determined by diffusion according to Fick's law and Stefan's law [25] , [26] , which are combined in the general expression for g smax given by equation (1) [27] (see Methods section). In this equation, Fick’s law relates the rate of steady-state diffusion to the concentration gradient across the stomatal pore, whereas Stefan's law describes the familiar ‘end correction’ component of the pore resistance [27] . As smaller stomata reduce the diffusion distance across the stomatal pore and limit the resistance of the ‘end correction’ term in equation (1), evolution towards higher g smax was necessarily linked to a reduction in stomatal size combined with an increase in stomatal density [24] ( Fig. 1c ). Coeval with this rise in g smax , the geologic record reveals a two-phased rise in angiosperm leaf vein density ( D v ) [14] , [15] during the Cretaceous ( Fig. 1d ). The first phase in rising angiosperm D v occurred around 100 Ma during the Late Albian [15] when, for the first time, the non-angiosperm maximum D v of ~6 mm mm −1 was surpassed. The second phase occurred in the latest Cretaceous and earliest Tertiary (around 60 Ma), during which the first modern values of angiosperm D v in excess of ~10 mm mm −2 are observed and angiosperm leaf gas exchange capacity escalated [15] . As a reference to the Cretaceous rise in angiosperm leaf venation, modern values of D v observed in woody shade demanders, in canopy trees and in extant megathermal rain forests are also indicated in Fig. 1d [15] . Although the evolution towards more reticulated leaf venation appears to have occurred on the backdrop of the Cretaceous C a decline ( cf. Fig. 1 ), relating rising angiosperm leaf venation to falling C a remains elusive [28] . Plant physiological modelling does suggest that the combined effect of higher D v and higher g smax may have enabled evolving angiosperms to increase leaf gas exchange rates to offset the adverse effects of falling C a for productivity [14] , [19] . However, to benefit from such highly conductive leaves in terms of additional growth and reproduction, the required additional carbon investments in water transport tissue should have been paid off by a larger increase in carbon gain [11] , [12] , [13] . On the basis of a combination of data and modelling approaches, we propose and substantiate a novel mechanism to explain why evolving angiosperms could suddenly expand their leaf gas exchange capacity during the Cretaceous, and why conifers could not. This proposed mechanism is based on the consequences of morphological differences between planar-shaped hypostomatous (angiosperm) broad leaves and tubular shaped (conifer) needle leaves for the leaf interior transport paths of CO 2 and water ( Fig. 1e ). We note that also non-angiosperm species evolved planar-shaped leaves with a variety venation structures [29] ; however, these morphologies did not evolve the high D v values common to modern upper canopy angiosperm species [14] , [15] , [20] . In our schematization of the broad-leaf morphology we differentiated between the Early Cretaceous angiosperm morphology with low D v and low D s and the modern angiosperm morphology with high D v and high D s . Common for all leaf morphologies is that CO 2 moves from the leaf boundary layer, through the stomatal pore and substomatal cavity into the intercellular airspaces [30] . From there, CO 2 is absorbed in the mesophyll cells where photosynthesis occurs in the chloroplasts [31] . Water moves from the soil through the plant’s water transport system up to the leaf veins before it evaporates and passes through the stomata. The exact mechanisms responsible for leaf interior water transport beyond the vein endings up to the stomata remain debated [32] , but may involve a liquid-phase flow through the apoplast, across individual cells and through plasmodesmata with evaporation occurring close to the stomata in the substomatal cavitiy. Alternatively, evaporation may occur deeper inside the leaf throughout the mesophyll [33] or close to the leaf vein endings [34] , [35] , with water being transported as a vapour across the intercellular airspaces up to the stomata. Recent advances highlight the importance of this vapour-phase water transport mechanism in regulating short-term stomatal responses [36] , [37] . Currently, neither the liquid-phase mechanism nor the vapour-phase mechanism can unambiguously be falsified [32] . Moreover, both water transport mechanisms may occur in parallel or involve a mixed phase [38] . We therefore explored the role of both mechanisms in relation to the sudden ecological success of angiosperms during the Cretaceous. We find that the period of rapid angiosperm evolution initiated after the leaf interior (post venous) transport path length for water became shorter than the leaf interior transport path length for CO 2 . This transition may have enabled the evolving angiosperms to develop leaves with higher gas exchange capacities required to adapt to the Cretaceous CO 2 decline and outcompete previously dominant coniferous species in the upper canopy. Postvenous liquid water transport and photosynthesis Considering the postvenous liquid-phase water transport mechanism, the maximum gas exchange capacity of a leaf is crucially constrained by its hydraulic conductance ( K leaf ) and the maximal leaf water potential gradient (Δ ψ leaf ) before tissue damage and hydraulic failure occurs [20] . A key determinant in K leaf is the maximum path length for postvenous water transport ( ( l H 2 O( l ) ) ). As shown in Fig. 2a , a log-linear relation exists between ( l H 2 O( l ) ) and K leaf across species [20] . An important consequence of the evolutionary rise in angiosperm D v was therefore the reduction in ( l H 2 O( l ) ) by bringing the leaf vein endings closer to the stomatal pores ( Fig. 2b ). The physiological advantage of the high D v in modern angiosperms is likely to be related to facilitating leaf water transport within the range of permissible Δ ψ leaf (ref. 20 ) before stomata close to protect plants from hydraulic failure [39] . The rise in D v may therefore have provided evolving angiosperms with a means to offset a rising transpirational demand associated with higher stomatal conductance and the functioning in environments with lower atmospheric humidity, such as the upper canopy. The relation between D v and stomatal conductance under variable atmospheric humidity is illustrated in Fig. 2c using a semi-empirical model [14] . This model assumes steady-state equilibrium between the liquid flux of water through the leaf interior up to the substomatal cavity, and the transpiration flux of water vapour through the stomata. The potential maximum photosynthetic carbon return from this water flux was calculated with the biochemical demand model of Farquhar et al . [40] This calculation involved the assumption that stomatal conductance to water vapour ( g sw ) equals stomatal conductance to CO 2 ( g sc ) when compensated for the difference in diffusivity between water vapour and CO 2 (that is, g sw = α · g sc , with α =1.6). Although leaf venation is not the only determinant in linking leaf water transport to photosynthesis [14] , [20] , the modelled values of g sw ( Fig. 2c ) imply that rising D v may have enabled evolving angiosperms to sustain photosynthesis under increasingly low atmospheric humidity and under falling C a ( Fig. 2d ). These results indicate that the sudden rise in angiosperm D v that occurred during the Cretaceous was related to their coeval radiation from the forest floor towards the upper canopy [4] . However, as shown previously by Boyce and Zwieniecki [28] using the same semiempirical model based on the liquid-phase mechanism [14] , there appears to be little carbon uptake advantage from increasing D v beyond ~8 mm mm −2 . Other mechanisms are therefore required to explain why angiosperm leaf venation evolved so suddenly beyond 6–10 mm mm −2 during the Late Cretaceous. 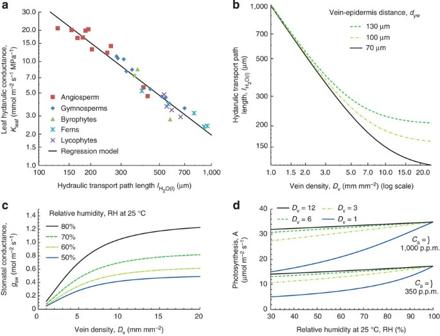Figure 2: Postvenous liquid water transport path length and leaf gas exchange rates. (a) Log-linear relation betweenlH2O(l)and the leaf hydraulic conductance (Kleaf) across species. Data are derived from Brodribbet al.20and includes observations on angiosperms, gymnosperms, byrophytes, ferns and lycophytes. Gymnosperm species with accessory transfusion tissue were omitted. A highly significant quadratic regression describing these data is:Kleaf=0.259lH2O(l)2+1.41lH2O(l)+0.60 (r2=0.94,P<0.001). (b) Geometric relation betweenDvandlH2O(l). Calculations show differences in vein-epidermis distance (dyw) covering a typical range of 70–130 μm (refs5,14,20). (c) Calculations with a semiempirical model14that relatesKleafto the stomatal conductance to water vapour (gsw) under steady-state transpiration with variableDv. The role of risingDvin allowing higher gswbecomes more apparent under lower atmospheric humidity owing to higher atmospheric demand. Relative atmospheric humidity (RH) was calculated for a constant temperature of 25 °C. (d) Calculations with the semiempirical model14under steady-state transpiration and steady-state photosynthesis rates (A) with variable atmospheric humidity (expressed as RH at a constant 25 °C) and variableDv. The stomatal conductance to CO2(gsc) was calculated under the assumption thatgsw=α·gscwithα=1.6. Simulations were performed for approximate modern and CretaceousCaof 350 and 1,000 p.p.m., respectively. Figure 2: Postvenous liquid water transport path length and leaf gas exchange rates. ( a ) Log-linear relation between l H 2 O( l ) and the leaf hydraulic conductance ( K leaf ) across species. Data are derived from Brodribb et al . [20] and includes observations on angiosperms, gymnosperms, byrophytes, ferns and lycophytes. Gymnosperm species with accessory transfusion tissue were omitted. A highly significant quadratic regression describing these data is: K leaf =0.259 l H 2 O( l ) 2 +1.41 l H 2 O( l ) +0.60 ( r 2 =0.94, P <0.001). ( b ) Geometric relation between D v and l H 2 O( l ) . Calculations show differences in vein-epidermis distance ( d yw ) covering a typical range of 70–130 μm (refs 5 , 14 , 20 ). ( c ) Calculations with a semiempirical model [14] that relates K leaf to the stomatal conductance to water vapour ( g sw ) under steady-state transpiration with variable D v . The role of rising D v in allowing higher g sw becomes more apparent under lower atmospheric humidity owing to higher atmospheric demand. Relative atmospheric humidity (RH) was calculated for a constant temperature of 25 °C. ( d ) Calculations with the semiempirical model [14] under steady-state transpiration and steady-state photosynthesis rates (A) with variable atmospheric humidity (expressed as RH at a constant 25 °C) and variable D v . The stomatal conductance to CO 2 ( g sc ) was calculated under the assumption that g sw = α · g sc with α =1.6. Simulations were performed for approximate modern and Cretaceous C a of 350 and 1,000 p.p.m., respectively. Full size image Leaf interior distances for CO 2 and water vapour transport To provide an answer to the question why evolving angiosperms so suddenly increased their leaf gas exchange capacity by increasing D v beyond the Late Cretaceous maximum, we involve a role for leaf interior water vapour transport in relation to leaf interior CO 2 transport. Hereto we calculated the maximum path length for water vapour transport between the leaf vein ending and the stomatal pore (termed the l H 2 O( g ) ), and the maximum path length for leaf interior CO 2 transport (termed the l CO 2 ). In contrast to the liquid-phase water transport mechanism discussed previously, this approach is based on the mechanism that water evaporates deep inside the mesophyll close to the leaf vein endings [34] , [35] , [36] and that CO 2 experiences an additional resistance by travelling between the stomatal pore and the sites of carboxylation [41] . When considering this vapour-phase mechanism, the relative distances of l H 2 O( g ) and l CO 2 are important because they influence the rate of water vapour and CO 2 transport through the intercellular airspaces, and thereby provide a mechanism to alter the tradeoff between water loss and carbon gain. Moreover, diffusion around individual stomata inside the leaf is a three-dimensional process, whereby the driving concentration gradients are altered both by the length of the diffusion path and by the size of the stomatal pore [30] . At the basis of our vapour-phase model were our calculations of evolutionary changes in l H 2 O( g ) relative to l CO 2 that occurred in angiosperms and conifers during the Cretaceous. For this analysis we used reconstructed ranges in D v and D s for Cretaceous angiosperms ( Fig. 1d and Supplementary Table S1 , respectively) and the schematised leaf morphologies of broad-leaved angiosperms and needle-leaved conifers ( Fig. 1e ). We note that also leaf thickness is relevant for determining the l H 2 O( g ) and l CO 2 , however, this plant trait is problematic to infer from compressed fossil material [5] . We therefore assumed typical ranges in vein-epidermal distance of 70–130 μm, as commonly applied for modelling leaf gas exchange of Cretaceous species [5] , [14] . Details on these calculations are presented in the Supplementary Methods . Our analysis of l H 2 O( g ) relative to l CO 2 revealed that a fundamental transition may have occurred in angiosperm leaf evolution at the onset of their global radiation. The critical D v at which l H 2 O( g ) = l CO 2 ranges from 2.5–5 mm mm −2 , depending on vein-epidermal distance and D s ( Fig. 3a ). The D v of modern canopy angiosperms in excess of 5 mm mm −2 ( cf. Fig. 1d (refs 14 , 15 )) therefore exceeds this critical D v . Hence, l H 2 O( g ) is shorter than l CO 2 in densely veined modern angiosperms. In contrast, the D v of Early Cretaceous angiosperms of ~1–6 mm mm −2 (refs 5 , 14 , 15 ) lies on or below this critical D v . Following the evolution in angiosperm leaf venation based on ancestral-state analyses [14] for an intermediate vein-epidermal distance of 100 μm indicated that l H 2 O( g ) became shorter than l CO 2 before the onset of the angiosperm radiation during the Early Cretaceous ( Fig. 3b ). Using observations on fossil angiosperm D v [15] for the same calculation revealed a similar pattern that is somewhat delayed relative to ancestral state reconstruction. These fossil data indicated that before the onset of the angiosperm radiation (before 110 Ma), the average l H 2 O( g ) was longer than l CO 2 , with an average ratio in l H 2 O( g ) / l CO 2 of 1.14 (with standard error of mean, s.e.m.=0.024). At the onset of the escalating rise in angiosperm D v (between 105 and 98 Ma) the average l H 2 O( g ) became shorter than l CO 2 , with an average ratio in l H 2 O( g ) / l CO 2 of 0.80 (s.e.m.=0.005). This development continued during the latest Cretaceous and earliest tertiary (77–58 Ma) when l H 2 O( g ) was reduced even further to an average ratio in l H 2 O( g ) / l CO 2 of 0.62 (s.e.m.=0.003). A similar shift did not occur in the schematised needle leaf as l H 2 O( g ) remained longer than l CO 2 due to its central-veined and tubular morphology ( Supplementary Fig. S1 ). 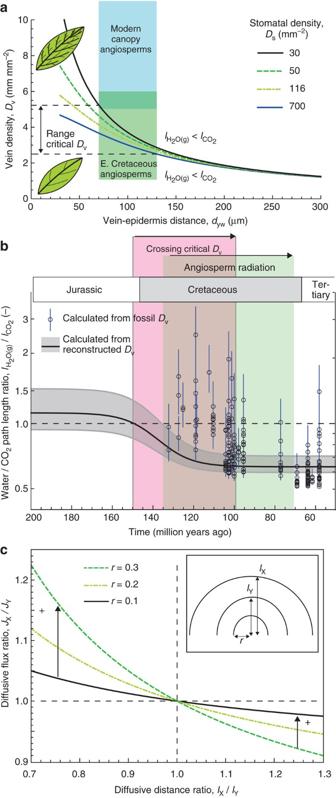Figure 3: Relative distances of leaf interior CO2and water (vapour) transport. (a) Calculation of the criticalDvfor whichlH2O(l)equalledlCO2in the schematised angiosperm leaf morphology. Calculation of the criticalDvusedDsin a range of 30–700 mm−2as observed in extant relatives of Early Cretaceous angiosperms5and assuming a typical range in vein-epidermal distance (dyw) of 70 and 130 μm (refs5,14). Dashed lines indicate crossing of the criticalDvat ~2.5–5 mm mm−2. Approximate ranges ofDvobserved in Early Cretaceous angiosperms (1–6 mm mm−2) and modern canopy angiosperms (>5 mm mm−2) (refs5,14,15) are indicated. (b) Evolutionary changes in the ratiolH2O(l)/lCO2through time. Calculations are based on angiospermDvobtained from fossil leaves15(circles with error bars) and age-calibrated ancestral-state analyses (grey sigmoid curve)14. The calculations assumed an average Early Cretaceous angiospermDsof 116 mm−2(Supplementary Table S1) and a range indywof 70–130 μm (refs5,14,20), with a highlighted intermediate value of 100 μm. The dashed line indicates the critical ratiolH2O(l)/lCO2=1. Crossing of this critical ratio occurred during the Early Cretaceous at the onset of the angiosperm radiation. AveragelH2O(g)/lCO2values calculated fromDvobserved on fossil leaves15assuming an intermediatedywof 100 μm for three crucial stages in angiosperm leaf vein evolution are: 1.14 (with s.d., σ=0.36 withn=30 observations) for 132–110 Ma, 0.80 (σ=0.23,n=95) for 105–98 Ma, and 0.62 (σ=0.13, n=90) for 77–58 Ma. Time ranges of these stages are based on the timing of the two-phased escalation of angiospermDv15. (c) Surpassing the criticalDvpotentially allowed evolving angiosperms to optimize leaf gas exchange and experience a carbon uptake advantage by reducing stomatal pore size. The proposed mechanism is shown by the theoretical relation between diffusive fluxes of substances X and Y (JXandJY) relative to their respective radial diffusion distances (lXandlY) from a single hemispherical pore with variable radiusr(equation (14))42. Figure 3: Relative distances of leaf interior CO 2 and water (vapour) transport. ( a ) Calculation of the critical D v for which l H 2 O( l ) equalled l CO 2 in the schematised angiosperm leaf morphology. Calculation of the critical D v used D s in a range of 30–700 mm −2 as observed in extant relatives of Early Cretaceous angiosperms [5] and assuming a typical range in vein-epidermal distance ( d yw ) of 70 and 130 μm (refs 5 , 14 ). Dashed lines indicate crossing of the critical D v at ~2.5–5 mm mm −2 . Approximate ranges of D v observed in Early Cretaceous angiosperms (1–6 mm mm −2 ) and modern canopy angiosperms (>5 mm mm −2 ) (refs 5 , 14 , 15 ) are indicated. ( b ) Evolutionary changes in the ratio l H 2 O( l ) / l CO 2 through time. Calculations are based on angiosperm D v obtained from fossil leaves [15] (circles with error bars) and age-calibrated ancestral-state analyses (grey sigmoid curve) [14] . The calculations assumed an average Early Cretaceous angiosperm D s of 116 mm −2 ( Supplementary Table S1 ) and a range in d yw of 70–130 μm (refs 5 , 14 , 20 ), with a highlighted intermediate value of 100 μm. The dashed line indicates the critical ratio l H 2 O( l ) / l CO 2 =1. Crossing of this critical ratio occurred during the Early Cretaceous at the onset of the angiosperm radiation. Average l H 2 O ( g ) / l CO 2 values calculated from D v observed on fossil leaves [15] assuming an intermediate d yw of 100 μm for three crucial stages in angiosperm leaf vein evolution are: 1.14 (with s.d., σ=0.36 with n =30 observations) for 132–110 Ma, 0.80 (σ=0.23, n =95) for 105–98 Ma, and 0.62 (σ=0.13, n=90) for 77–58 Ma. Time ranges of these stages are based on the timing of the two-phased escalation of angiosperm D v [15] . ( c ) Surpassing the critical D v potentially allowed evolving angiosperms to optimize leaf gas exchange and experience a carbon uptake advantage by reducing stomatal pore size. The proposed mechanism is shown by the theoretical relation between diffusive fluxes of substances X and Y ( J X and J Y ) relative to their respective radial diffusion distances ( l X and l Y ) from a single hemispherical pore with variable radius r (equation (14)) [42] . Full size image We hypothesize that surpassing the critical D v gave evolving angiosperms a competitive advantage over conifers when falling C a required rising g smax via increases in D s and decreases in stomatal pore size. Key to the proposed mechanism is that the tradeoff between CO 2 transport and water vapour transport through the leaf interior is altered by differences in l CO 2 and l H 2 O( g ) and, considering the three-dimensionality of diffusion, the size of the stomatal pore. This mechanism is illustrated for the diffusive fluxes of two conceptual substances ( J X , J Y ) with equal diffusivity (assumed unity) driven by an equal concentration difference (also assumed unity) over different radial distances ( l X and l Y ) from a single hemispherical pore with variable radius ( r ) ( Fig. 3c ), according to equation (14) (ref. 42 ). The first result shown by this example is that the diffusive flux is highest of that substance, which diffuses over the shortest radial distance. Interpreting this first result for leaf interior fluxes of CO 2 and water vapour around individual stomata indicates that the highest carbon flux relative to a water vapour flux can be achieved when l CO 2 is shorter than l H 2 O( g ) . This situation would resemble the diffusion distances in the schematised conifer and early angiosperm leaf morphologies ( cf. Fig. 1e ). The second result of this example is that a change in pore radius has the largest effect on the flux of the substance that diffuses over the shortest radial distance. The physiological implication of this second result is that when l H 2 O( g ) < l CO 2 , as in the schematised modern angiosperm leaf morphology, a decrease in pore size leads to a larger decrease in leaf interior water vapour transport than in CO 2 transport. On the basis of this mechanism, we propose that when angiosperms surpassed the critical D v (which rendered l H 2 O( g ) < l CO 2 ) they could increase leaf interior CO 2 transport relative to leaf interior water vapour transport by developing leaves with more and smaller stomatal pores. The consequences of developing leaves with more and smaller stomata not only affected leaf interior gas transport, but also allowed evolving angiosperms to increase g smax due to the combined implications of Fick’s law and Stefan’s law. Hence, gradually surpassing the critical D v may have suddenly created an opportunity for evolving angiosperms to increase their stomatal gas exchange capacity. Leaf interior water vapour transport and photosynthesis We investigated the hypothesized vapour-phase mechanism with an analytical model of leaf gas exchange, which coupled the diffusion pathways of CO 2 and water vapour between the atmosphere and the stomata to their respective diffusion pathways in the leaf interior. A graphical representation of our model approach is shown in Supplementary Fig. S2 . We thereby considered the schematised morphologies of needle-leaved conifers and broad-leaved angiosperms ( Fig. 1e ) to calculate the ratio in l H 2 O( g ) / l CO 2 resulting from changes in D v and D s . To reveal the subsequent consequences of changes in stomatal pore size and D s for leaf gas exchange, we solved the model for maximum photosynthetic carbon returns from equal transpirative water loss assuming that water evaporates deep inside the mesophyll near the leaf vein endings [34] , [35] , [36] . This analysis was based on the premise that the maximum water transport capacity of the whole plant constrains the maximum transpiration rate, which in turn determines maximum photosynthesis and productivity in a specific evaporative environment [20] . Further details on our model approach, including the assumptions and an evaluation with empirical data, are provided in the Supplementary Methods . Our model showed that the conifer and Early Cretaceous angiosperm leaf morphologies (with l H 2 O( g ) > l CO 2 ) permit relatively high photosynthesis with equal water loss due to the relatively short distance for CO 2 transport and the relatively large distance for water transport inside the leaf ( Fig. 4a ). A rise in D s combined with a decrease in stomatal pore size led to diminishing carbon returns with equal water loss for these leaf morphologies. The combined values of D s and stomatal pore size (expressed as pore radian, r p ) used in these simulations are shown in Fig. 4b . In contrast, the angiosperm leaf morphology with D v beyond the critical density (thus with l H 2 O( g ) < l CO 2 ) appeared relatively inefficient with low D s but it may increase photosynthesis with equal water loss by developing leaves with higher D s and smaller pores. This carbon uptake advantage emerges from the model because, due to the three-dimensional character of diffusion, a development of smaller stomata most strongly reduces the flux of that substance which diffuses over the shortest radial distance around each single pore inside the leaf ( Fig. 3c ). As we solved our model for an equal water flux, the reduction in stomatal pore size was accompanied by an increase in D s ( Fig. 4b ). Important here is to consider that the same values of stomatal pore size and D s also govern the diffusion of CO 2 from the atmosphere into the leaf whereas l CO 2 does not, a priori , equal l H 2 O( g ) . Hence, the total leaf conductance to CO 2 ( g tc ), which includes both the stomatal and leaf interior conductance to CO 2 , is not, a priori , equal to g tw / α . Consequentially, our model revealed that depending on the ratio l H 2 O( g ) / l CO 2 , different carbon returns from equal water loss may be found as a function of stomatal pore size and D s under otherwise equal boundary conditions. 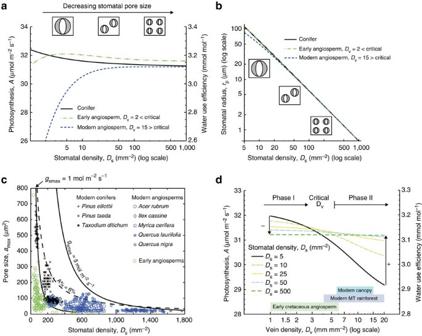Figure 4: A link between stomatal traits and leaf venation. (a) Simulated changes in maximum photosynthesis (A) with equal water loss for the conifer, and the early and modern angiosperm leaf morphologies as a function of stomatal density (Ds). Water use efficiency (WUE) is indicated on the second y axis. Changes inDsare associated with inverse changes in stomatal pore size to answer a constant water loss of 10 mmol m−2s−1. Depending on leaf morphology andDv, changes inDsand stomatal pore size have different effects ongicandgiw,and thereby affect the tradeoff between water loss and carbon gain. Simulations used constantCaof 1,000 p.p.m. and a constant relative atmospheric humidity of 80% at 25 °C as boundary conditions. (b) Relation betweenDsand stomatal pore size (expressed as pore radian,rp) in the simulated stomatal morphologies shown ina. (c) Relation betweenDsand the pore size of fully opened stomata (amax) observed in modern angiosperms (blue symbols) and modern conifers (black symbols) from Florida43and extant relatives of early angiosperms (green symbols)5. Lines of equal maximal stomatal conductance (gsmax) and leaf surface area allocated to fully opened stomatal pores (A%) are indicated. (d) Simulations of the vapour-phase mechanism suggest that angiosperms experienced a shift from falling (phase I) to rising (phase II) photosynthesis with equal water loss by increasingDsand reducingrpafter surpassing the criticalDv. WUE is indicated on the second y axis. Ranges ofDvobserved in Early Cretaceous and modern angiosperms15are also indicated to show that the simulated transition from phase I to phase II matches the divergence observed between Early Cretaceous and modern angiosperm leaf venation. Model boundary conditions are as described fora. Figure 4: A link between stomatal traits and leaf venation. ( a ) Simulated changes in maximum photosynthesis ( A ) with equal water loss for the conifer, and the early and modern angiosperm leaf morphologies as a function of stomatal density ( D s ). Water use efficiency (WUE) is indicated on the second y axis. Changes in D s are associated with inverse changes in stomatal pore size to answer a constant water loss of 10 mmol m −2 s −1 . Depending on leaf morphology and D v , changes in D s and stomatal pore size have different effects on g ic and g iw, and thereby affect the tradeoff between water loss and carbon gain. Simulations used constant C a of 1,000 p.p.m. and a constant relative atmospheric humidity of 80% at 25 °C as boundary conditions. ( b ) Relation between D s and stomatal pore size (expressed as pore radian, r p ) in the simulated stomatal morphologies shown in a . ( c ) Relation between D s and the pore size of fully opened stomata ( a max ) observed in modern angiosperms (blue symbols) and modern conifers (black symbols) from Florida [43] and extant relatives of early angiosperms (green symbols) [5] . Lines of equal maximal stomatal conductance ( g smax ) and leaf surface area allocated to fully opened stomatal pores ( A % ) are indicated. ( d ) Simulations of the vapour-phase mechanism suggest that angiosperms experienced a shift from falling (phase I) to rising (phase II) photosynthesis with equal water loss by increasing D s and reducing r p after surpassing the critical D v . WUE is indicated on the second y axis. Ranges of D v observed in Early Cretaceous and modern angiosperms [15] are also indicated to show that the simulated transition from phase I to phase II matches the divergence observed between Early Cretaceous and modern angiosperm leaf venation. Model boundary conditions are as described for a . Full size image This result revealed that with l H 2 O( g ) < l CO 2 , as in the modern angiosperm leaf morphology, a reduction in pore size combined with an increase in D s may have increased the CO 2 flux relative to an equal water vapour flux. As evolution will likely have favoured those individuals that achieve highest carbon returns within the constraint of the whole-plant water transport capacity, we expect to find evidence for the proposed mechanism in observations of D s and stomatal pore sizes on the leaves of conifers, early angiosperms and modern angiosperms. We therefore compared observations of these stomatal traits of modern conifers and angiosperms from the mid to upper canopy of subtropical forests in Florida [43] with observations on extant relatives of Early Cretaceous angiosperms [5] ( Fig. 4c ). Statistical comparisons of stomatal traits between these groups are presented in Supplementary Table S1 . These data indicated that modern angiosperms develop leaves with most and smallest stomata of the three groups. The differences in these stomatal properties also showed that the modern angiosperms profit most from the combined implications of Fick's law and Stefan's law and reach highest g smax . This advantage of developing leaves with many small stomata is illustrated by the solid and dashed lines in Fig. 4c , indicating equal g smax and the percentage of leaf surface allocated to fully opened stomatal pores ( A % ), respectively. A sudden carbon uptake advantage for evolving angiosperms The proposed ability of angiosperms that surpassed the critical D v to profit from developing leaves with more and smaller stomata provides a mechanism to explain the revolutionary escalation of angiosperm leaf gas exchange during the Cretaceous. In accordance with fossil evidence [15] , the proposed mechanism entails that angiosperm evolution occurred in two phases with the first phase linked to D v rising up to the critical density, and a second phase during which their gas exchange capacity escalated. During the first evolutionary phase, our model revealed that highest carbon returns from equal water loss could be achieved with few and large stomata ( Fig. 4d ). The second phase started when surpassing the critical D v rendered l H 2 O( g ) < l CO 2 . From that moment onwards, our model revealed that evolving angiosperms could increase photosynthesis with equal water loss by developing leaves with more and smaller stomata. Moreover, the influence of stomatal traits on modelled carbon uptake became larger with higher D v , which indicates a functional benefit from increasing D v beyond the Cretaceous maximum of 6–10 mm mm −2 . We propose that surpassing the critical D v may therefore have facilitated evolving angiosperms to develop leaves with more and smaller stomata and more reticulated venation, whereas coniferous species remained to develop less densely veined leaves with relatively few and large stomata. An important concept for the interpretation of these results is the idea that water loss presents a cost to plants. As a result, short-term changes in stomatal aperture are aimed at the optimization of carbon gain with minimal water loss [44] , [45] depending on environmental conditions [46] . The optimization hypothesis may also explain the adaptation of the stomatal traits governing g smax at decadal [23] or at evolutionary timescales [47] . On the basis of our results we propose to expand the concept of optimal gas exchange to describe the adjustments of stomatal pore size and D s in relation to evolutionary adaptations in leaf morphology and venation. Similar to the observations on stomatal traits shown in Fig. 4b , our vapour-phase model suggests that conifers and early angiosperms (with l H 2 O( g ) > l CO 2 ) may optimize minimal water loss with maximum carbon gain by developing leaves with relatively few and large stomata rather than leaves with more and smaller stomata. Our results also indicate that angiosperms that surpassed the critical D v (with l H 2 O( g ) < l CO 2 ) could optimize the tradeoff between carbon uptake and water loss by developing leaves with more and smaller stomata, permitting higher g tc within the constraint of A % ( Fig. 5a ). As a result of this gas exchange advantage, we propose that angiosperms with D v beyond the critical density experienced a competitive advantage over angiosperms with lower D v and coniferous species when an increase g tc was required to prevent carbon ‘starvation’ [19] during the Cretaceous C a decline ( Fig. 5b ). Although these results are based on the concept that water is transported (partly) as a vapour through the intercellular airspaces [34] , [35] , [36] , [37] , rising D v likely also facilitated liquid-phase leaf water transport [14] , [20] . Potentially, the liquid and vapour-phase mechanisms may have acted in concert, whereby crossing the critical D v initiated an evolutionary development towards higher g smax and higher K leaf . However, the liquid-phase mechanism alone does not provide a clear explanation for the sudden escalation of angiosperm D v beyond the Cretaceous maximum of ~6–10 mm mm −2 (ref. 28 ). 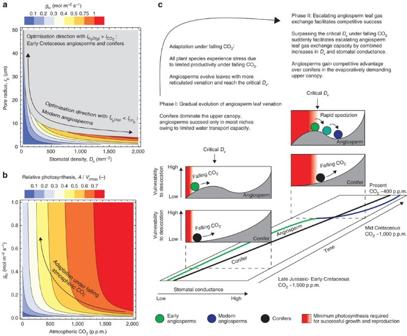Figure 5: Evolutionary changes in stomatal and venation traits during the Cretaceous. (a) Relations between stomatal density (Ds), stomatal pore radius (rp) and total leaf conductance to CO2(gtc). Proposed directions of stomatal trait optimization are indicated. Values ofgtcthat require >10% of the leaf surface to be allocated to fully opened stomatal pores (A%) are shaded grey. Highestgtccan only be achieved within the constraint of thisA%by developing leaves with highDsand smallrp. Constant relative atmospheric humidity of 80% at 25 °C was used as boundary condition. (b) FallingCarequired a rise ingtcto sustain photosynthesis rates (A). TheAis scaled relative to maximum carboxylation rate (Vcmax) as changes inVcmaxlikely occurred at geological timescales19. Atmospheric humidity is as ina. (c) Conceptual overview of how crossing of the criticalDvfacilitated the Cretaceous angiosperm revolution. Key to the proposed mechanism is that leaf venation and stomatal gas exchange are intrinsically linked20, and that rising stomatal conductance increases the vulnerability to desiccation unless a more extensive leaf water transport system can answer the additional water flux32. As angiosperms exhibited a sudden increase in leaf venation after surpassing the criticalDv, their vulnerability to desiccation (as indicated by the grey surfaces) shows a hump-shaped relationship over time. In contrast, conifers experienced a steady increase in their vulnerability to desiccation as their leaf water transport system evolved only marginally through time14. We suggest that the first phase in angiosperm leaf vein evolution gradually drove angiosperm leaf evolution to a maximum in vulnerability to desiccation. Surpassing the criticalDvthen suddenly enabled evolving angiosperms to increase carbon returns from (equal) water loss by developing leaves with more and smaller stomata resulting in higher stomatal conductance. This development facilitated evolving angiosperms to invest in expanding leaf water transport tissue to reduce their vulnerability to desiccation and increase productivity in drier atmospheres, such as the upper canopy. The resulting competitive advantage of angiosperms over conifers may explain their competitive success and rapid speciation during the Cretaceous1,6,7,8. Figure 5: Evolutionary changes in stomatal and venation traits during the Cretaceous. ( a ) Relations between stomatal density ( D s ), stomatal pore radius ( r p ) and total leaf conductance to CO 2 ( g tc ). Proposed directions of stomatal trait optimization are indicated. Values of g tc that require >10% of the leaf surface to be allocated to fully opened stomatal pores ( A % ) are shaded grey. Highest g tc can only be achieved within the constraint of this A % by developing leaves with high D s and small r p . Constant relative atmospheric humidity of 80% at 25 °C was used as boundary condition. ( b ) Falling C a required a rise in g tc to sustain photosynthesis rates ( A ). The A is scaled relative to maximum carboxylation rate ( V cmax ) as changes in V cmax likely occurred at geological timescales [19] . Atmospheric humidity is as in a . ( c ) Conceptual overview of how crossing of the critical D v facilitated the Cretaceous angiosperm revolution. Key to the proposed mechanism is that leaf venation and stomatal gas exchange are intrinsically linked [20] , and that rising stomatal conductance increases the vulnerability to desiccation unless a more extensive leaf water transport system can answer the additional water flux [32] . As angiosperms exhibited a sudden increase in leaf venation after surpassing the critical D v , their vulnerability to desiccation (as indicated by the grey surfaces) shows a hump-shaped relationship over time. In contrast, conifers experienced a steady increase in their vulnerability to desiccation as their leaf water transport system evolved only marginally through time [14] . We suggest that the first phase in angiosperm leaf vein evolution gradually drove angiosperm leaf evolution to a maximum in vulnerability to desiccation. Surpassing the critical D v then suddenly enabled evolving angiosperms to increase carbon returns from (equal) water loss by developing leaves with more and smaller stomata resulting in higher stomatal conductance. This development facilitated evolving angiosperms to invest in expanding leaf water transport tissue to reduce their vulnerability to desiccation and increase productivity in drier atmospheres, such as the upper canopy. The resulting competitive advantage of angiosperms over conifers may explain their competitive success and rapid speciation during the Cretaceous [1] , [6] , [7] , [8] . Full size image Considering the proposed vapour-phase mechanism, a positive feedback in angiosperm leaf evolution may emerge from the combined adaptations of stomatal traits and leaf venation because additional carbon uptake can increase growth and productivity. These additional carbon gains may have been invested in expanding leaf water transport tissue to sustain growing transpiration rates. In contrast, if rising stomatal conductance is not supported by an increase in water transport capacity, plants become more vulnerable to desiccation [32] . The initial phase of gradual leaf vein evolution, potentially related to reducing the carbon cost associated with developing an extensive water transport system [12] , [13] , may therefore have suddenly facilitated the rapid evolution of angiosperm leaf venation beyond the critical D v [14] , [15] . The resulting escalation in leaf gas exchange capacity likely permitted evolving angiosperms to leave their original moist niches near the dark forest floor [4] , [5] , and become more successful in the drier and brighter upper canopy [8] . To interpret crossing of the critical D v as a critical transition [48] , we argue that gradually reducing l H 2 O( g ) beyond l CO 2 provided angiosperms with a sudden carbon uptake advantage over coniferous species during the Cretaceous C a decline [17] . As light, CO 2 and water are key resources for all plants, the sudden increase in angiosperm leaf gas exchange capacity during the Cretaceous C a decline may explain their rapid speciation in niches previously dominated by conifers [49] . Surpassing the critical D v is therefore proposed to have been the pivotal moment that facilitated the evolutionary rise of angiosperms towards modern biodiversity. This critical transition in angiosperm leaf evolution is shown conceptually in Fig. 5c . Although crossing of the critical D v may explain the sudden rise in angiosperm leaf gas exchange capacity, the question remains why a similar evolution did not occur in other clades that also evolved planate leaves with diverse venation structures [20] , [29] . As leaves with many small stomata and highly reticulated venation provide a clear carbon uptake advantage under low C a [14] , [24] , novel insights may be obtained by unravelling the mechanisms that prevented non-angiosperm clades from evolving these leaf traits. Stomatal size, density and conductance relations The maximal stomatal conductance to water vapour ( g smax ) and to CO 2 ( g cmax ) (both with units mol m −2 s −1 ) were calculated from stomatal properties as [24] : and where D H 2 O and D CO 2 (m 2 s −1 ) are diffusivities of water vapour and CO 2 , respectively, v (m 3 mol −1 ) is the molar volume of air, D s is stomatal density (m −2 ), a max is stomatal pore size with fully inflated guard cells (m 2 ) and p d (m) is pore depth. The a max was calculated from measurements of pore length assuming stomata are ellipse-shaped with pore width equal to half the pore length [43] . The p d was calculated from species-specific relations with guard cell width for the modern conifers and angiosperms from Florida [23] , [43] and based on measurements for extant relatives of Early Cretaceous angiosperms [5] . When g smax was calculated to visualize the scaling with D s and a max (for example Fig. 4b ), the species average relation between guard cell width and p d for the modern conifers and angiosperms was used [23] . The percentage of the leaf surface area occupied by fully opened stomatal pores ( A % ) was calculated as: Photosynthesis Steady-state photosynthetic carbon returns ( A 1 (mol m −2 s −1 )) were calculated with the biochemical model of Farquhar et al . [40] in both the liquid and the gas phase model: where C i is the leaf interior CO 2 concentration (mol mol −2 ), c p is the CO 2 compensation point (mol mol −1 ) and the a 1 (mol m −2 s −1 ) and a 2 (mol mol −1 ) are determined by whether photosynthesis is limited by light or by Rubisco. As we assume maximum photosynthesis rates (light saturation), a 1 equals the maximum carboxylation capacity . Here, K c (mol mol −1 ) and K o (mol mol −1 ) are the Michaelis constants for CO 2 fixation and oxygen inhibition, respectively, and the C oa (mol mol −1 ) is the oxygen concentration in the air. For values of these parameters and their temperature dependencies, we followed Katul et al . [45] , hence K c was assumed 300 μmol mol −1 , K o was assumed 300 mmol mol −1 and C oa was assumed 210 mmol mol −1 at a temperature of 25 °C. A constant V cmax value of 59 mol m −2 s −1 was assumed to represent the maximum carboxylation rate at 25 °C. We note that up and down regulation of V cmax likely occurred in response to changes in C a [19] and that altered oxygen levels also affected photosynthesis during the Cretaceous [50] , [51] . Yet, we assumed constant photosynthesis parameters to allow testing our hypothesis on the effect of stomatal and leaf morphological adaptations on leaf gas exchange. Liquid-phase model Our simulations for liquid-phase water transport were based on a previously published semiempirical model [14] . This model was parameterized for a broad variety of species, including extant relatives of Early Cretaceous angiosperms, modern angiosperms and conifers [14] , [20] . The model relates leaf vein density ( D v (mm mm −2 )) to the length of postvenous liquid apoplastic water flow path ( l H 2 O ( l ) (μm)), leaf hydraulic conductance ( K leaf (mmol MPa −1 m −2 s −1 )) and actual stomatal conductance to water vapour ( g sw (mol m −2 s −1 ) according to the following set of equations: The leaf internal water transport distance parallel to the plane of the leaf ( d xw (l) (μm)) was calculated as [14] : in which the empirically derived value of 650 accounts for the hierarchical pattern of leaf venation in angiosperm broad leaves [14] , [20] . The vein-epidermal distance perpendicular to the plane of the leaf ( d yw (μm)) was assumed to be in the range of 70–130 μm, following previous plant physiological modelling work [5] , [14] , [20] , [28] . The curvature (or turtuosity) of the liquid flow path through the leaf interior ( τ ) was assumed π/2 following Brodribb et al . [20] For the maximum permissible leaf water potential gradient ( Δψ leaf ) we assumed a value of 0.4 MPa, following Brodribb and Feild [14] . Further, to calculate the difference in water vapour content between the leaf boundary layer ( w a (mol mol −1 )) and the substomatal cavity ( w s (mol mol −1 )) we assumed saturation at 25 °C. Assuming steady-state so that the transpirative water vapour flux ( E 1 (mol m −2 s −1 )) equals leaf interior liquid water flow ( E 2 (mol m −2 s −1 ), equations (5, 6, 7, 8, 9) can be combined as: A second expression for the potential maximum photosynthetic carbon return ( A 2 (mol m −2 s −1 )) was calculated from equation (10) under the assumption that g sw = α · g sc, with : Here, C a and C i are the CO 2 concentrations in the atmosphere and inside the leaf (mol mol −1 ), respectively. With C i being the only unknown in two expressions for carbon uptake (equations 4 and 11), the steady-state photosynthesis rate was obtained by iteratively solving the expression A 1 = A 2 using the software Wolfram Mathematica 7.0 to find the correct C i with a prescribed C a . Vapour-phase model To solve the equations for leaf gas exchange in our vapour-phase model we simplified equations (1) and (2) by assuming that stomata had circular shapes with radius ( r p ) and p d equal to ½ r p : and It should be noted that stomata are sometimes ellipse or dumbbell-shaped [52] , which could potentially alter g smax related to a specific pore length. However, also in these cases diffusion through stomata remains governed by Fick’s law and Stefan's law yielding a similar relation between pore size, D s and g smax [26] , [53] . Consideration of alternative stomatal shapes would therefore not fundamentally alter our results. We simulated leaf interior transport of CO 2 and water vapour around individual stomata by using the analytical solution of three-dimensional spherical diffusion [42] . This solution describes the three-dimensional diffusive flux J (mol s −1 ) of a substance with diffusivity D (m 2 s −1 ) from a single (hemi)spherical pore with radius r (m) over a radial distance l (m) driven by a concentration difference between the pore interior C 1 (mol mol −1 ) and the concentration C 2 (mol mol −1 ) at radial distance l : The basic results of this equation were presented in Fig. 3c to indicate the scaling of diffusive fluxes of two comparable substances over different distances around a single hemispherical pore of variable size. The three-dimensional solution for the conductance g 3D (mol s −1 ) over a radial distance ( l ) from a single hemispherical pore with radius ( r) may then be written as: Prior modelling results [30] have indicated that the concentration gradients around the end of the stomatal pore in the leaf interior take the form of a hemisphere with a radius approximately equal to r p . Expanding on these results, we assumed that the CO 2 and water vapour concentrations at the end of the stomatal pore equalled the concentrations at the start/end of their respective leaf interior diffusion pathways. Hereby we note that the ‘end correction’ term to account for these spherical diffusion shells around individual stomata was applied to both sides of the stomatal pore in equations 12 and 13 (ref. 27 ). Hence, we extended the analytical solution of g 3D to represent multiple stomata expressed per unit leaf surface area to simulate the leaf interior conductance of CO 2 ( g ic (mol m −2 s −1 )) between the end of the stomatal pore and the sites of carboxylation as: where l CO 2 (m) represents the maximum radial diffusion distance for CO 2 , η (−) accounts for part of the leaf interior CO 2 transport occurring through the mesophyll cells [30] , and θ (−) and τ (−) denote the porosity and tortuosity of the leaf interior assumed to be ½ and π/2, respectively. Our calculation of l CO 2 and the estimation of the parameter η are presented in the Supplementary Methods . Similar to the calculation of g ic , we calculated the leaf interior (postvenous) conductance of water vapour g iw (mol m −2 s −1 ) over the maximum distance between the leaf vein endings and the stomatal pore l H 2 O( g ) (m) as: Our calculation of l H 2 O( g ) is also presented in the Supplementary Methods . Assuming conservation of mass, the respective transport pathways of CO 2 and water vapour across the stomata and through the leaf interior were coupled. This allowed us to express stomatal conductance and leaf interior conductance as a series of resistances, which may be summed up to a single total conductance to CO 2 ( g tc (mol m −2 s −1 )): and a total conductance to water ( g tw (mol m −2 s −1 )): in which f d (−) is a constant compensating for the difference between the geometric maximal stomatal conductance and the actual stomatal conductance during periods of maximum photosynthesis. We assumed f d to be ½ representing plants functioning at a Δψ leaf that initiates a 50% reduction in actual stomatal conductance [39] . The CO 2 transport from the atmosphere to the sites of carboxylation inside the leaf ( A 3 (mol m −2 s −1 )) was then calculated as: and water vapour transport from the leaf vein endings to the atmosphere E 3 (mol m −2 s −1 ) was calculated as: The w i (mol mol −1 ) represented the water vapour concentration in the intercellular airspaces near the leaf vein endings, for which we assumed saturation at a constant temperature of 25 °C. To obtain the results presented in Fig. 4a , a fixed maximum transpiration rate ( E 3 ) of 10 mmol m −2 s −1 was expressed in terms of g tw assuming a constant atmospheric relative humidity of 80% with temperature of 25 °C. As both g tw and g tc are functions of the variables D s and r p (equations 18 and 19), we expressed g tw in terms of those D s and r p required to answer the specified E 3 (equation 21). With C i being the only unknown in two expressions for carbon uptake (equations 4 and 20), the steady-state photosynthesis rate was obtained from iteratively solving the expression A 1 = A 3 by finding the correct C i using the software Wolfram Mathematica 7.0. Photosynthesis could then be expressed as a function of D s and, for the angiosperm leaf morphology, also as a function of D v . We note that solving our model for higher constant transpiration rates yielded higher values of g tw , which also yielded higher photosynthesis rates for all leaf morphologies. How to cite this article: de Boer H. J. et al . A critical transition in leaf evolution facilitated the Cretaceous angiosperm revolution. Nat. Commun. 3:1221 doi: 10.1038/ncomms2217 (2012).